Jarid2 is induced by TCR signalling and controls iNKT cell maturation Jarid2 is a reported component of three lysine methyltransferase complexes, polycomb repressive complex 2 (PRC2) that methylates histone 3 lysine 27 (H3K27), and GLP-G9a and SETDB1 complexes that methylate H3K9. Here we show that Jarid2 is upregulated upon TCR stimulation and during positive selection in the thymus. Mice lacking Jarid2 in T cells display an increase in the frequency of IL-4-producing promyelocytic leukemia zinc finger (PLZF) hi immature invariant natural killer T (iNKT) cells and innate-like CD8 + cells; Itk-deficient mice, which have a similar increase of innate-like CD8 + cells, show blunted upregulation of Jarid2 during positive selection. Jarid2 binds to the Zbtb16 locus, which encodes PLZF, and thymocytes lacking Jarid2 show increased PLZF and decreased H3K9me3 levels. Jarid2-deficient iNKT cells perturb Th17 differentiation, leading to reduced Th17-driven autoimmune pathology. Our results establish Jarid2 as a novel player in iNKT cell maturation that regulates PLZF expression by modulating H3K9 methylation. Covalent modifications of histone tails, such as acetylation, methylation and phosphorylation, are critical for chromatin function [1] . Active promoters and enhancers are generally marked by histone H3 lysine 4 (H3K4) methylation, transcribed genes by H3K36me3 trimethylation (H3K36me3) and inactive promoters by H3K27me3 or H3K9me3 (ref. 2 ). The H3K27me3 modification is generated by polycomb repressive complex 2 (PRC2), a lysine methyltransferase complex that contains three core subunits, Ezh2, Suz12 and Eed (ref. 3 ). PRC2 proteins play a central role in embryonic development and regulate many biological processes in the adult, including lymphopoiesis, cell cycle and X chromosome inactivation [4] , [5] . Loss of PRC2 components results in aberrant differentiation of pluripotent embryonic stem cells (ESCs) [6] , and several Polycomb group genes have been identified as oncogenes or tumour suppressors [4] . Recent studies have identified Jarid2 (also known as Jumonji, Jmj), the founding member of the JmjC domain-containing protein family, as a novel component of PRC2 (refs 7 , 8 , 9 , 10 , 11 ). Jarid2 lacks the conserved residues essential for histone demethylase activity and hence is predicted to be catalytically inactive [12] . Jarid2 is also reported to be part of a G9a- and GLP-containing protein complex that promotes H3K9 methylation on the cyclin D1 promoter [13] and silences the expression of cyclin D1 and other cell cycle genes [14] . Moreover, Jarid2 is a direct binding partner of SETDB1 (SET domain, bifurcated 1 protein) in developing heart tissue and is essential for the recruitment of SETDB1 to the Notch1 locus, and di- and trimethylation of H3K9 at this locus, resulting in Notch1 silencing [15] . Jarid2 is critical for embryonic development. Jarid2-deficient (Jmj−/−) mouse embryos display diverse developmental defects [16] . To study the importance of histone modifications in biological processes, several groups have focused on T-cell development in the thymus and T-cell differentiation into effector cells in the periphery [17] , [18] , [19] . The development of mature T-cell receptor (TCR) αβ-positive T cells in the thymus is largely regulated by signals received from the TCR and/or accessory proteins such as costimulatory or cytokine receptors. Weak or no signals result in death by neglect, whereas moderate signals lead to positive selection and the consequent development of mature CD4 and CD8 single positive (SP) thymocytes [20] . Strong signals, as from agonist peptides, prompt the deletion of TCR-expressing cells or—in a process termed agonist selection [20] —divert them to alternate cell fates. These alternate cell lineages include NKT cells, H2-M3-restricted cells, CD8αα intraepithelial lymphocytes and CD4 + CD25 + regulatory T cells. Each of these lineages is selected in the thymus, each has important roles in regulating normal immune responses and each requires a different degree of signalling through the TCR [21] , [22] . NKT cells are a well-characterized subset of T cells that bear CD1d-restricted αβ TCRs: in mice, the TCRs combine an invariant Vα14-Jα18 rearrangement of the α-chain with Vβ8, Vβ7 or Vβ2 β-chains; in humans, a TCRα chain with a homologous invariant Vα24-Jα18 rearrangement is paired with a Vβ11 β-chain [23] . These cells, generally referred to as invariant NKT cells (iNKT cells), are distinct from other T cells that express NK receptors, and from T cells with more diverse receptors that recognize CD1d. iNKT cells are derived from CD4 + CD8 + double positive (DP) precursors [24] but their developmental pathway subsequently diverges from that of mainstream T cells. As this specific TCRαβ rearrangement is rare, iNKT cells are normally present at very low levels in TCR + DP thymocytes. However, probably because the semi-invariant TCR expressed by iNKT cells recognizes various self- and microbial lipid-containing antigens, rare iNKT cell precursors undergo massive expansion in the thymus on interaction with ligands presented by CD1d on other DP cells, and subsequently acquire an effector phenotype along with receptors of the NK cell lineage; homotypic interactions through SLAM family proteins expressed by DP cells are also involved [23] . The effector functions of iNKT cells are characterized by the peculiar ability to rapidly release both interleukin (IL)-4 and interferon-γ (IFN-γ) without priming [23] , although more specialized iNKT cell subsets, such as those devoted to IL-17A synthesis [25] , have also been described. PLZF (encoded by Zbtb16 ) is a signature transcription factor of the iNKT cell lineage. PLZF directs the iNKT cell effector programme, specifying the migratory properties of iNKT cells and the ability to produce cytokines immediately upon stimulation [26] , [27] . Mutations in Zbtb16 abrogate the memory-effector properties of iNKT cells, resulting in their reversal to a naive phenotype and their redistribution to the lymph nodes rather than to the liver and other organs where they normally predominate. Constitutive expression of PLZF at physiological levels during thymic development induces an effector programme in all conventional T cells, independently of their antigen specificity [28] . Egr2, one of the earliest transcriptional factors induced by TCR signalling, directly binds and activates the Zbtb16 promoter, resulting in PLZF expression and providing a link between TCR signalling and cell fate determination in the thymus [29] . We examined the role of Jarid2 in T-cell development and function, based on our observation that Jarid2 mRNA is rapidly upregulated in stimulated T cells [30] . We show that Jarid2 is upregulated after positive selection in the thymus, and that mice with a conditional deletion of Jarid2 in the T-cell compartment express increased levels of PLZF in DP thymocytes and display abnormal iNKT cell development. The iNKT cells in these mice have an immature (or iNKT2) phenotype and influence other T-cell populations, both in the thymus and in the periphery. Chromatin immunoprecipitation (ChIP) assays demonstrated direct binding of Jarid2 to the PLZF ( Zbtb16 ) promoter in DP cells, and DP cells lacking Jarid2 show decreased levels of the repressive H3K9me3 modification at the PLZF ( Zbtb16 ) locus. The similar phenotype of increased iNKT and innate CD8 T cells was observed in inducible T-cell kinase-2 (Itk2)-deficient mice with blunted upregulation of Jarid2 during positive selection, supporting a model in which deficient TCR signalling leads to decreased expression of Jarid2, which in turn leads to increased expression of PLZF and broad effects on systemic immunity. Our data identify Jarid2 as a key transcriptional repressor that restricts iNKT cell commitment by linking TCR signalling to H3K9me3 modification and repression of PLZF. Jarid2 expression is induced on TCR activation Stimulation of CD4 + T cells with anti-CD3 and anti-CD28 led to a rapid increase in Jarid2 mRNA ( Fig. 1a ) and protein ( Fig. 1b and Supplementary Fig. 1a ), corroborating our previous finding that Jarid2 mRNA is rapidly upregulated in stimulated T cells [30] . The discordance between low mRNA and high protein levels at 20–24 h ( Fig. 1a,b and Supplementary Fig. 1a ) suggests post-transcriptional regulation of Jarid2 protein levels, potentially through miRNAs. Analysis of DP thymocytes showed that Jarid2 mRNA levels increased from the CD69 − to the CD69 + stage, indicating that Jarid2 expression is also induced by TCR stimulation during thymocyte-positive selection ( Fig. 1c ). 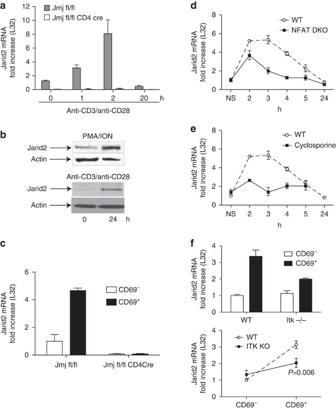Figure 1: Jarid2 is induced upon TCR stimulation. (a,d,e) Naive CD4+T cells were purified from spleen and lymph nodes of the indicated mice, and restimulated with plate bound anti-CD3/anti-CD28 antibodies for the indicated times. Total RNA was obtained and Jarid2 and ribosomal L32 (as quantitative control for normalisation) mRNA expression was measured by RT qReal-time PCR (qPCR). (b) Spleen and lymph nodes were harvested from C57BL/6 (B6) mice, and CD4+T cells were purified and restimulated with PMA/Ionomycin or anti-CD3/anti-CD28 for 24 h. Total protein extracts were purified and Jarid2 or β-Actin protein expression was determined by western blot. (candf) CD69−(pre-positive selection) or CD69+(post-positive selection) DP (CD4+CD8+) thymocytes were purified by fluorescence-activated cell sorting (FACS) fromJmj fl/flandJmj fl/fl CD4Cre(c) or WT B6 andItk−/−mice (f). Total RNA was purified and Jarid2 and ribosomal L32 mRNA expression were measured by qPCR. All experiments were repeated at least twice. With exception of the bottom panel inf, error bars are calculated from qPCR triplicates and are representative of at least two independent experiments. Inf, the top panel shows the result for one pair of WT andItk−/−mice and is representative of three different pairs. The bottom panel represents the three different pairs of WT andItk−/−mice combined (two independent experiments). The fold change for all the pairs was analysed by unpairedt-test. Error bars show mean and s.e.m. of three replicates in the same experiment. Except forfbottom, all the graphics show one experiment representative of at least two completely independent experiments. WT, wild type C57BL/6 (B6); NFAT DKO,NFAT1−/− NFAT2 fl/fl CD4Cre. Figure 1: Jarid2 is induced upon TCR stimulation. ( a , d , e ) Naive CD4 + T cells were purified from spleen and lymph nodes of the indicated mice, and restimulated with plate bound anti-CD3/anti-CD28 antibodies for the indicated times. Total RNA was obtained and Jarid2 and ribosomal L32 (as quantitative control for normalisation) mRNA expression was measured by RT qReal-time PCR (qPCR). ( b ) Spleen and lymph nodes were harvested from C57BL/6 (B6) mice, and CD4 + T cells were purified and restimulated with PMA/Ionomycin or anti-CD3/anti-CD28 for 24 h. Total protein extracts were purified and Jarid2 or β-Actin protein expression was determined by western blot. ( c and f ) CD69 − (pre-positive selection) or CD69 + (post-positive selection) DP (CD4 + CD8 + ) thymocytes were purified by fluorescence-activated cell sorting (FACS) from Jmj fl/fl and Jmj fl/fl CD4Cre ( c ) or WT B6 and Itk−/− mice ( f ). Total RNA was purified and Jarid2 and ribosomal L32 mRNA expression were measured by qPCR. All experiments were repeated at least twice. With exception of the bottom panel in f , error bars are calculated from qPCR triplicates and are representative of at least two independent experiments. In f , the top panel shows the result for one pair of WT and Itk−/− mice and is representative of three different pairs. The bottom panel represents the three different pairs of WT and Itk−/− mice combined (two independent experiments). The fold change for all the pairs was analysed by unpaired t -test. Error bars show mean and s.e.m. of three replicates in the same experiment. Except for f bottom, all the graphics show one experiment representative of at least two completely independent experiments. WT, wild type C57BL/6 (B6); NFAT DKO, NFAT1−/− NFAT2 fl/fl CD4Cre . Full size image TCR stimulation results in calcium mobilization and consequent activation of Nuclear factor of activated T-cells (NFAT) transcription factors [31] . We used T cells doubly deficient in NFAT1 and NFAT2 to show that upregulation of Jarid2 mRNA depends, at least in part, on NFAT activation ( Fig. 1d,e ). Naive CD4 + T cells from Nfat1 −/− , Nfat2 fl/fl CD4Cre (NFAT DKO) mice were activated in vitro with anti-CD3/CD28 for different times, and Jarid2 mRNA levels were analysed by quantitative real-time PCR (qPCR). Induction of Jarid2 expression on TCR activation was strongly reduced in doubly NFAT-deficient cells ( Fig. 1d ); the residual upregulation may reflect the presence of NFAT4, a third NFAT family member present in immune cells. NFAT is activated by the phosphatase calcineurin, which dephosphorylates multiple phosphoserines in the regulatory domain of NFAT, leading to NFAT nuclear translocation [31] . Consistent with involvement of the calcineurin-NFAT pathway [30] , Jarid2 upregulation in response to TCR stimulation was repressed by the calcineurin inhibitor cyclosporine A ( Fig. 1e ). The Tec family tyrosine kinases Itk and Rlk are required for Ca 2+ mobilization and PLC-γ1 phosphorylation/activation following stimulation of the TCR [32] . Itk−/− and double Rlk−/− Itk−/− mice have multiple defects in T-cell development, cytokine production and T-helper cell differentiation [33] . CD8 + T cells from these mice show an ‘innate-like’ T-cell phenotype, defined by high expression of CD122, CD44, CXCR3 and Eomes, and the ability to produce IFN-γ immediately on stimulation [34] , [35] . As this phenotype resembled that of mice with Jarid2 deficiency in T cells (see below), we quantified Jarid2 mRNA levels in thymocytes of Itk−/− mice and wild-type (WT) controls pre- and post-positive selection. Indeed, although thymocytes from WT control mice showed a pronounced three- to four-fold increase of Jarid2 mRNA on positive selection ( Fig. 1f , also see Fig. 1c ), Itk−/− mice showed a significantly blunted response ( Fig. 1f ). The residual induction of Jarid2 mRNA in Itk -deficient thymocytes is likely to be due to compensation from other Tec kinases. Generation of innate CD8 + T cells in Jarid2-deficient mice To study the role of Jarid2 in T-cell development and function, we generated mice with a T cell-specific deficiency in Jarid2 by crossing mice homozygous for a conditional (floxed) allele of Jarid2 ( Jmj fl/fl ) [36] with CD4Cre mice. CD4 + T cells in spleen and lymph nodes of Jmj fl/fl CD4Cre mice completely deleted the floxed Jmj alleles and lacked Jarid2 mRNA and protein expression ( Figs 1a,c and 2a,b and Supplementary Fig. 1b,c ). Jmj fl/fl CD4Cre mice showed no significant change in total cell numbers in the spleen, thymus or lymph nodes ( Fig. 1c ), but showed an increase in the frequency of CD8 + SP (CD8 SP) thymocytes, without a significant difference ( P >0.05) in the total numbers of these cells ( Fig. 2d ). A high proportion of these CD8 SP cells were CD44 hi CD122 hi CXCR3 hi ( Fig. 2e,f ) and rapidly produced IFN-γ in response to TCR stimulation ( Fig. 2g ); a substantial fraction also expressed the T-box transcription factor Eomes, which is associated with the expression of CD122 (IL-2 and IL-15 receptor β-chain) and secretion of IFN-γ by memory CD8 + T cells [37] ( Fig. 2f ). 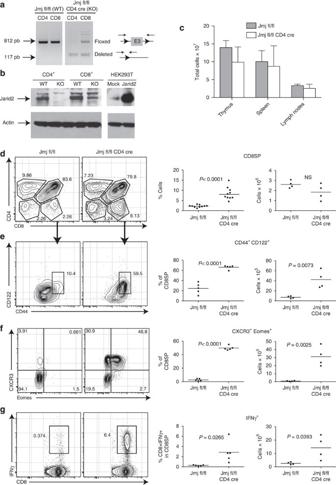Figure 2: Jarid2 deficiency leads to increased generation of innate CD8+T cells in the thymus. (a,b) CD4+and CD8+T cells isolated fromJmj fl/florJmj fl/fl CD4Cremice were stimulated with plate-bound anti-CD3/anti CD28 antibodies for an initial 72 h and expanded in the presence of IL-2 for an additional 3 days. (a) Genomic DNA was extracted and PCR was performed using primers flanking thefloxedJarid2 exon3. (b) Total protein was analysed by western blotting with antibodies specific for Jarid2 or β-actin. HEK293T cells overexpressing murine Jarid2 were used as control. (c) Thymi, spleens and lymph nodes were harvested fromJmj fl/florJmj fl/fl CD4Cremice and the total number of cells were counted using Accuri. Error bars show mean and s.d. (d–g) Flow cytometric analysis of thymocytes fromJmj fl/florJmj fl/fl CD4Cremice. (d) Shown is the frequency of CD4- and CD8-expressing cells. Each dot represents one mouse (of a total of ten mice from five independent experiments). Note the expanded population of CD8 SP thymocytes. Right, the percentage and numbers of CD8SP cells in individual mice are shown. Cells in the CD8 SP gate shown indwere analysed for CD122, CD44 (e), CXCR3 or Eomes (f) expression, and for IFN-γ production after PMA/ionomycin stimulation (g). Starting fromd,e, all the experiments were repeated at least four times. For all the graphics, each mouse is represented as one dot. Data were analysed by unpairedt-test. ns, not significant. Bars represent mean values for all the mice. Figure 2: Jarid2 deficiency leads to increased generation of innate CD8 + T cells in the thymus. ( a , b ) CD4 + and CD8 + T cells isolated from Jmj fl/fl or Jmj fl/fl CD4Cre mice were stimulated with plate-bound anti-CD3/anti CD28 antibodies for an initial 72 h and expanded in the presence of IL-2 for an additional 3 days. ( a ) Genomic DNA was extracted and PCR was performed using primers flanking the floxed Jarid2 exon3. ( b ) Total protein was analysed by western blotting with antibodies specific for Jarid2 or β-actin. HEK293T cells overexpressing murine Jarid2 were used as control. ( c ) Thymi, spleens and lymph nodes were harvested from Jmj fl/fl or Jmj fl/fl CD4Cre mice and the total number of cells were counted using Accuri. Error bars show mean and s.d. ( d – g ) Flow cytometric analysis of thymocytes from Jmj fl/fl or Jmj fl/fl CD4Cre mice. ( d ) Shown is the frequency of CD4- and CD8-expressing cells. Each dot represents one mouse (of a total of ten mice from five independent experiments). Note the expanded population of CD8 SP thymocytes. Right, the percentage and numbers of CD8SP cells in individual mice are shown. Cells in the CD8 SP gate shown in d were analysed for CD122, CD44 ( e ), CXCR3 or Eomes ( f ) expression, and for IFN-γ production after PMA/ionomycin stimulation ( g ). Starting from d , e , all the experiments were repeated at least four times. For all the graphics, each mouse is represented as one dot. Data were analysed by unpaired t -test. ns, not significant. Bars represent mean values for all the mice. Full size image Impaired iNKT cell maturation in Jarid2-deficient mice Mice deficient in or expressing mutant forms of diverse T-cell signalling molecules or transcription factors including the scaffold protein SLP-76 (ref. 38 ), Itk [34] , [35] , the transcription factor KLF2 (Krüppel-like factor 2) [39] , [40] , the histone acetyltransferase CBP (CREB-binding protein) [41] and the transcriptional regulator Id3 (inhibitor of DNA binding 3) [42] also display an increase in the frequency and numbers of innate CD8 + T cells (reviewed in ref. 43 ). Innate CD8 + T cells are barely detectable in WT C57BL/6 mice, and their presence in these mutant mice has been attributed to the expansion of small numbers of PLZF + IL-4-producing cells, including iNKT cells. As the CD8 SP thymocytes in Jarid2 -deficient mice resembled innate CD8 + T cells, we assessed the presence of iNKT cells in the thymus of these mice. Using CD1d α-GalCer tetramer staining to detect iNKT cells, we observed a decrease rather than an increase in the frequency and total number of iNKT cells in the thymus of Jmj fl/fl CD4Cre mice ( Fig. 3a ). A more comprehensive analysis revealed a defect in iNKT maturation ( Fig. 3b ). At least three stages of iNKT cell maturation in the thymus have been described: CD44 lo NK1.1 − naive cells (stage 1), CD44 hi NK1.1 − effector cells (stage 2) and terminally differentiated CD44 hi NK1.1 + cells (stage 3) ( Fig. 3b , left panel) [44] ; a newer classification into NKT1, NKT2 and NKT17 cells [45] is considered below. Whereas iNKT cells in the thymus of control Jmj fl/fl mice had largely matured to stage 3, iNKT cells in the thymus of Jmj fl/fl CD4Cre mice were arrested at the stage 2 to stage 3 transition, as the vast majority of cells were phenotypically stage 1 or stage 2 and expressed high levels of CD4 ( Fig. 3b , right panel). 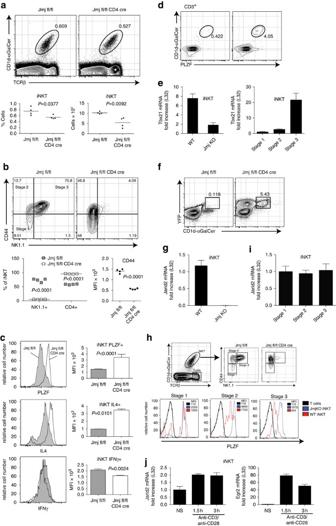Figure 3: Jarid2 deficiency in thymocytes results in expansion of PLZF+cells in the thymus and the periphery. iNKT cells are defined here as CD1d-αGalCer-tetramer+TCRβ+cells. (a) Representative histogram depicting iNKT cell frequencies in the thymus ofJmj fl/florJmj fl/fl CD4Cremice (top). Bottom panels, percentages and total numbers of iNKT cells in individual mice. (b) Expression of CD44 and NK1.1 on iNKT cells gated as inaand additionally on CD24−cells (not shown). Top, representative histogram depicting percentages of CD44+NK1.1+iNKT cells. Bottom, quantification with each dot representing one mouse: percentage of CD4+NK1.1+iNKT cells (left) or CD44 mean fluorescence intensity (MFI) in iNKT cells (right). (c) PLZF expression, IL-4 and IFN-γ production measured by intracellular staining in iNKT cells gated as ina. Error bars show mean and s.d. from four different mice in the same experiment. For cytokine production, thymocytes were stimulated with PMA/ionomycin. Right, results from four individual mice. All the data were analysed by non-pairedt-test. ns, nonsignificant. (d) Spleen and lymph nodes fromJmj fl/florJmj fl/fl CD4Cremice were stained for iNKT cell markers and PLZF. Plots are gated on CD3+B220−CD25−CD8−cells. (e)Tbx21(Tbet) and ribosomal protein L32 mRNA levels were analysed by quantitative real-time reverse transcription PCR (qRT–PCR) in RNA from sorted iNKT cells ofJmj fl/florJmj fl/fl CD4Cremice (left), and different stages of iNKT cells defined by staining with anti-CD44 and anti-NK1.1 (right). Error bars show mean of PCR triplicates and s.e.m. (f) Spleen and lymph node cells fromJmj fl/florJmj fl/flCD4Cre crossed toRosa26 YFP Sf/Sfreporter (R26R) mice were stained with the CD1d-αGalCer tetramer and analysed for YFP expression by flow cytometry. (g) iNKT cells from WT or Jarid2 KO thymocytes were sorted, andJarid2and ribosomal protein L32 mRNA levels were analysed by qRT–PCR. Error bars show mean of PCR triplicates and s.e.m. (h) PLZF expression was determined on thymic iNKT cells fromJmj fl/florJmj fl/fl CD4Cremice (gating strategy shown above), or conventional T cells (TCRβ+CD1d-αGalCer tetramer −) as controls. Numbers indicate MFI for PLZF at each stage of development. (i) Thymocytes from B6 orJmj fl/fl CD4Cremice were sorted for stages of iNKT development as inh, andJarid2and ribosomal protein L32 mRNA levels were analysed by qRT–PCR. (j) Sorted iNKT cells from B6 thymocytes were activated with αGalCer-pulsed DC, expandedin vitroin the presence of IL-7, and restimulated with anti-CD3/anti-CD28 after 14 days.Jarid2,Egr2and ribosomal protein L32 mRNA levels were analysed by qRT–PCR. Error bars show mean of PCR triplicates and s.e.m. The data are representative of three independent experiments ina,b,g, two independent experiments inc,d,hand one experiment ine,f,j. Figure 3: Jarid2 deficiency in thymocytes results in expansion of PLZF + cells in the thymus and the periphery. iNKT cells are defined here as CD1d-αGalCer-tetramer + TCRβ + cells. ( a ) Representative histogram depicting iNKT cell frequencies in the thymus of Jmj fl/fl or Jmj fl/fl CD4Cre mice (top). Bottom panels, percentages and total numbers of iNKT cells in individual mice. ( b ) Expression of CD44 and NK1.1 on iNKT cells gated as in a and additionally on CD24 − cells (not shown). Top, representative histogram depicting percentages of CD44 + NK1.1 + iNKT cells. Bottom, quantification with each dot representing one mouse: percentage of CD4 + NK1.1 + iNKT cells (left) or CD44 mean fluorescence intensity (MFI) in iNKT cells (right). ( c ) PLZF expression, IL-4 and IFN-γ production measured by intracellular staining in iNKT cells gated as in a . Error bars show mean and s.d. from four different mice in the same experiment. For cytokine production, thymocytes were stimulated with PMA/ionomycin. Right, results from four individual mice. All the data were analysed by non-paired t -test. ns, nonsignificant. ( d ) Spleen and lymph nodes from Jmj fl/fl or Jmj fl/fl CD4Cre mice were stained for iNKT cell markers and PLZF. Plots are gated on CD3 + B220 − CD25 − CD8 − cells. ( e ) Tbx21 (Tbet) and ribosomal protein L32 mRNA levels were analysed by quantitative real-time reverse transcription PCR (qRT–PCR) in RNA from sorted iNKT cells of Jmj fl/fl or Jmj fl/fl CD4Cre mice (left), and different stages of iNKT cells defined by staining with anti-CD44 and anti-NK1.1 (right). Error bars show mean of PCR triplicates and s.e.m. ( f ) Spleen and lymph node cells from Jmj fl/fl or Jmj fl/fl CD4Cre crossed to Rosa26 YFP Sf/Sf reporter (R26R) mice were stained with the CD1d-αGalCer tetramer and analysed for YFP expression by flow cytometry. ( g ) iNKT cells from WT or Jarid2 KO thymocytes were sorted, and Jarid2 and ribosomal protein L32 mRNA levels were analysed by qRT–PCR. Error bars show mean of PCR triplicates and s.e.m. ( h ) PLZF expression was determined on thymic iNKT cells from Jmj fl/fl or Jmj fl/fl CD4Cre mice (gating strategy shown above), or conventional T cells (TCRβ + CD1d-αGalCer tetramer −) as controls. Numbers indicate MFI for PLZF at each stage of development. ( i ) Thymocytes from B6 or Jmj fl/fl CD4Cre mice were sorted for stages of iNKT development as in h , and Jarid2 and ribosomal protein L32 mRNA levels were analysed by qRT–PCR. ( j ) Sorted iNKT cells from B6 thymocytes were activated with αGalCer-pulsed DC, expanded in vitro in the presence of IL-7, and restimulated with anti-CD3/anti-CD28 after 14 days. Jarid2 , Egr2 and ribosomal protein L32 mRNA levels were analysed by qRT–PCR. Error bars show mean of PCR triplicates and s.e.m. The data are representative of three independent experiments in a , b , g , two independent experiments in c , d , h and one experiment in e , f , j . Full size image Several studies have demonstrated that immature iNKT cells in stages 1 and 2 express higher levels of PLZF compared with more mature iNKT cells [26] , [27] , and are more potent producers of IL-4 (refs 46 , 47 ). An alternative view is that some of these tetramer + but NK1.1-negative cells are not immature, but are fully differentiated to a so-called NKT2 subset that responds to IL-25 and that preferentially produces Th2 cytokines [48] . In concordance with these studies, we found that iNKT cells in the thymus of Jmj fl/fl CD4Cre mice expressed higher levels of PLZF compared with control Jmj fl/fl iNKT cells and also expressed relatively low levels of CD44, suggesting that they were to some extent immature; however, they also produced increased levels of IL-4 (but not IFN-γ) on phorbol-12-myristate-13-acetate (PMA)/ionomycin stimulation, consistent with skewing to a more NKT2 phenotype ( Fig. 3c ). We also observed an increase in the frequency of tetramer + PLZF + cells in the spleen ( Fig. 3d ). Consistent with the fact that Jarid2-deficient iNKT cells cannot proceed to stage 3 of development, we observed reduced levels of Tbx21 mRNA (encoding Tbet) in these cells ( Fig. 3e , left). Cells defined as stage 3 ( Fig. 3b ) possess the same phenotype as the recently defined NKT1 cells: CD44 hi NK1.1 + PLZF low with high levels of Tbet (ref. 45 and Fig. 3e , right). More detailed analyses will be needed to determine how Jarid2-deficient cells fit in the new proposed classification, but based on our data an alternative view is that Jarid2-deficient iNKT cells are preferentially NKT2 and do not differentiate properly into NKT1. To confirm that Jarid2 was indeed deleted in iNKT cells, we bred Jmj fl/fl or Jmj fl/fl CD4Cre mice to Rosa26 YFP Sf/Sf reporter mice (R26R). These mice possess a floxed STOP cassette preceding the yellow fluorescent protein (YFP) gene, whose excision permits YFP expression. In Jmj fl/fl CD4Cre R26R mice, essentially all iNKT cells defined by staining with Cd1d α-GalCer tetramer were YFP + ( Fig. 3f ), showing that Cre-mediated deletion occurred efficiently in the iNKT cell population. The deletion of Jarid2 was also confirmed at the mRNA level in sorted iNKT cells ( Fig. 3g ). The presence of innate CD8 + T cells in the thymus also correlates with the expansion of PLZF-positive γδ T cells [39] , [42] , but we did not observe any clear change in the frequency or numbers of these cells in thymocytes from Jmj fl/fl CD4Cre mice compared with controls ( Supplementary Fig. 2 ). Jmj fl/fl CD4Cre mice also displayed an increase in the frequency of iNKT cells in peripheral lymphoid tissues—spleen and lymph nodes—compared with control mice ( Fig. 4 ). As in the thymus, most of the iNKT cells in the spleen and lymph nodes of Jmj fl/fl CD4Cre mice were immature, displaying low levels of NK1.1 and CD44, and higher levels of CD4 ( Fig. 4a,b ). In non-lymphoid peripheral tissues—liver and lung—even though we saw increased frequencies of iNKT cells in the Jmj fl/fl CD4Cre mice, there was a less striking effect on the expression of maturation markers ( Fig. 4c,d ). 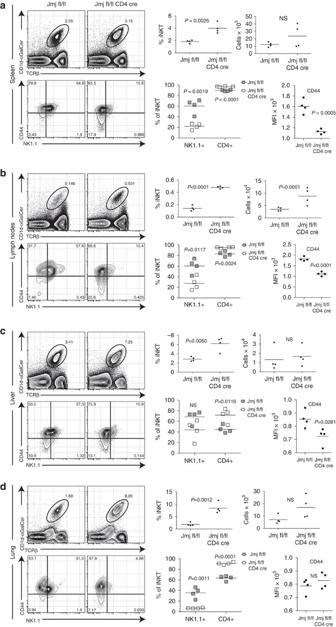Figure 4: Immature iNKT cells are expanded in the periphery of T cell Jarid2-deficient mice. Cells were obtained from the spleen (a), lymph nodes (b), liver (c) or lung (d) ofJmj fl/florJmj fl/fl CD4Cremice as indicated, and stained with CD1d-αGalCer tetramer or antibodies to CD44, NK1.1 and CD4. For each organ, the gates in the top graph represent total iNKTs. In the bottom graphs, cells were gated on CD1d-αGalCer tetramer+PLZF+cells (iNKTs). The data are representative of two independent experiments. In the graphs showing % or number of cells, each individual mouse is represented by a dot and the data were analysed by non-pairedt-test. NS, not significant. Figure 4: Immature iNKT cells are expanded in the periphery of T cell Jarid2-deficient mice. Cells were obtained from the spleen ( a ), lymph nodes ( b ), liver ( c ) or lung ( d ) of Jmj fl/fl or Jmj fl/fl CD4Cre mice as indicated, and stained with CD1d-αGalCer tetramer or antibodies to CD44, NK1.1 and CD4. For each organ, the gates in the top graph represent total iNKTs. In the bottom graphs, cells were gated on CD1d-αGalCer tetramer + PLZF + cells (iNKTs). The data are representative of two independent experiments. In the graphs showing % or number of cells, each individual mouse is represented by a dot and the data were analysed by non-paired t -test. NS, not significant. Full size image Jarid2 and Egr2 counter-regulate PLZF expression The increased levels of PLZF could be caused by a direct effect of Jarid2 on activation of the PLZF (Zbtb16) gene or could merely reflect an increased frequency of iNKT cells stuck at stages 1 and 2. To address this point, we stained iNKT cells at stages 1, 2 and 3 of development for PLZF expression ( Fig. 3h , top panel). The mean fluorescence intensity of PLZF staining was increased at all stages ( Fig. 3h , bottom panel), ruling out the possibility that the increase in PLZF levels is secondary to the accumulation of cells in stage 1 and 2, but consistent with the hypothesis that Jarid2 directly regulates PLZF (Zbtb16) expression. When we analysed mRNA obtained from sorted cells representing stages 1, 2 and 3 using the gating strategy shown in Fig. 3h , top panel, there was no clear change in Jarid2 mRNA levels between developmental stages ( Fig. 3i ), although a change in protein levels cannot be ruled out. In contrast, Zbtb16 mRNA and PLZF protein expression correlate positively with levels of Egr2 expression, as previously shown [29] ; moreover, the ~80-fold upregulation of Egr2 mRNA expression observed in iNKT cells on anti-CD3/anti-CD28 stimulation is much higher than the ~2-fold increase in Jarid2 mRNA expression under the same conditions ( Fig. 3j ). Together, these results indicate that Egr2 is the major positive determinant of PLZF (Zbtb16) expression at early developmental stages, whereas Jarid2 fine-tunes PLZF (Zbtb16) levels at later stages through a subsidiary suppressive role. Cell-intrinsic and -extrinsic effects of Jarid2 deficiency To ask whether Jarid2 deletion is associated with a cell-intrinsic defect in the maturation of iNKT cells, we set up mixed bone marrow chimeras in which a 1:1 mixture of CD45.2 + Jmj fl/fl or Jmj fl/fl CD4Cre progenitors and CD45.1 + WT B6 progenitors was transferred to irradiated Thy1.1 + mice ( Fig. 5a ). Flow cytometry analyses, gating on CD45.2 + CD1d α-GalCer tetramer + thymocytes, demonstrated that CD45.2 + iNKTs derived from Jmj fl/fl CD4Cre mice displayed a maturation defect ( Fig. 5b ) similar to that observed in Jmj fl/fl CD4Cre mice ( Fig. 3b ), while iNKTs cells derived from the control CD45.1 + population showed normal maturation phenotypes ( Fig. 5b ). This result indicates that the defect in iNKT development is a cell-intrinsic consequence of Jarid2 deletion in the precursors of iNKT cells in the thymus. On the other hand, development of innate CD8 + cells was observed in both in CD45.2 + and CD45.1 + subpopulations; this cell-extrinsic effect ( Fig. 5c ) is consistent with previous observations that immature iNKT PLZF hi cells drive the generation of innate CD8 + cells [35] , [39] , [43] , [49] . 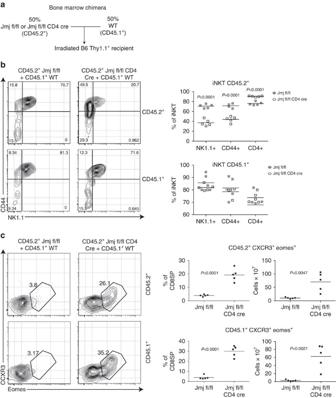Figure 5: The defect in iNKT maturation in Jarid2-deficient mice is cell intrinsic and the generation of innate CD8+ T cells is cell extrinsic. (a) Schematic representation of the mixed bone marrow chimera analysed inbandc. WT CD45.1+bone marrow cells were mixed in a 1:1 ratio with CD45.2+bone marrow cells from the indicated genotypes, then transferred into irradiated Thy1.1+congenic mice. Nine weeks after cell transfer, thymocytes were obtained and analysed by flow cytometry. (b) Stages of iNKT development determined by CD44 and NK1.1 staining. Top panel, cells were gated on controlJmj fl/fl(left) or Jarid2-deficientJmj fl/fl CD4Cre(right) CD45.2+iNKT cells (CD1d-αGalCer tetramer+TCRβ+Thy1.1−); bottom panel, cells were gated on the WT CD45.1+cells in the same chimeric mouse. Each plot is representative of five different mice. The scatter plots to the right depict the expression of the indicated iNKT maturation markers on individual mice. (c) The generation of innate CD8+T cells was analysed. Top panel, cells were gated on controlJmj fl/fl(left) or Jarid2- deficientJmj fl/fl CD4Cre(right) CD45.2+CD8 SP Thy1.1− cells; bottom panel, cells were gated on WT CD45.1+CD8 SP Thy1.1− cells. Cells were analysed for the expression of innate CD8+T cell markers: CXCR3 (surface) and eomes (intracellular). Each plot is representative of five different mice. The scatter plots to the right depict the frequency and total number of CXCR3+eomes+CD8 cells in individual mice. Data were analysed by unpairedt-test. NS, not significant. Figure 5: The defect in iNKT maturation in Jarid2-deficient mice is cell intrinsic and the generation of innate CD8+ T cells is cell extrinsic. ( a ) Schematic representation of the mixed bone marrow chimera analysed in b and c . WT CD45.1 + bone marrow cells were mixed in a 1:1 ratio with CD45.2 + bone marrow cells from the indicated genotypes, then transferred into irradiated Thy1.1 + congenic mice. Nine weeks after cell transfer, thymocytes were obtained and analysed by flow cytometry. ( b ) Stages of iNKT development determined by CD44 and NK1.1 staining. Top panel, cells were gated on control Jmj fl/fl (left) or Jarid2-deficient Jmj fl/fl CD4Cre (right) CD45.2 + iNKT cells (CD1d-αGalCer tetramer + TCRβ + Thy1.1 − ); bottom panel, cells were gated on the WT CD45.1 + cells in the same chimeric mouse. Each plot is representative of five different mice. The scatter plots to the right depict the expression of the indicated iNKT maturation markers on individual mice. ( c ) The generation of innate CD8 + T cells was analysed. Top panel, cells were gated on control Jmj fl/fl (left) or Jarid2- deficient Jmj fl/fl CD4Cre (right) CD45.2 + CD8 SP Thy1.1− cells; bottom panel, cells were gated on WT CD45.1 + CD8 SP Thy1.1− cells. Cells were analysed for the expression of innate CD8 + T cell markers: CXCR3 (surface) and eomes (intracellular). Each plot is representative of five different mice. The scatter plots to the right depict the frequency and total number of CXCR3 + eomes + CD8 cells in individual mice. Data were analysed by unpaired t -test. NS, not significant. Full size image Jarid2-deficient iNKT cells suppress Th17 differentiation iNKT cells profoundly influence autoimmune disease outcomes through their ability to rapidly express pro- and anti-inflammatory cytokines that influence the type and magnitude of the immune response [50] . Experimental autoimmune encephalomyelitis (EAE) in mice is a useful animal model for one such autoimmune condition, multiple sclerosis in humans. iNKT cells play an important modulatory role in EAE [50] , [51] , and the protective effects of α-GalCer against EAE require IL-4 and IL-10 secretion by iNKTs [51] . To address whether the abnormal development of iNKTs in Jmj fl/fl CD4Cre mice could affect the immune responses of other T cells in vivo , we used the myelin oligodendrocyte glycoprotein (MOG)-induced model of EAE ( Fig. 6a , left). The results showed a protective effect of Jarid2 deficiency in T cells, with reduced disease incidence ( Fig. 6a , middle) and less severe paralysis symptoms ( Fig. 6a , right). 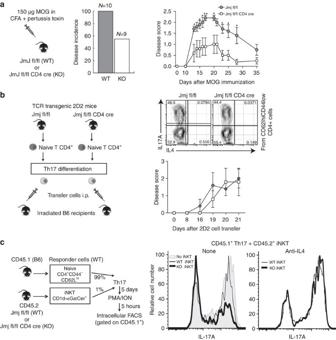Figure 6: Even a small contamination with Jarid2-deficient iNKT cells compromises Th17 differentiation. (a)Jmj fl/florJmj fl/fl CD4Cremice were immunized on day 0 with MOG(35–55) peptide in complete Freund’s adjuvant (CFA) and pertussis toxin (PTX) was administered intraperitoneally on days 0 and 1. Mice were monitored for neurological signs of EAE. Disease incidence in two combined independent experiments (middle panel); clinical scores (mean values±s.d.) in one representative experiment with at least four mice per group (right panel) are displayed. EAE disease scores were analysed by two way analysis of variance. **P<0.01, *P<0.05. (b) CD4+CD62Lhi, CD44lo(naive) T cells were isolated from 2D2 TCR-transgenic mice specific for MOG(35–55) peptide and stimulated in Th17-biasing conditions (IL-1β, IL-6 and IL-23) for 5 days. Cells were restimulated with plate-bound anti-CD3/anti-CD28 antibodies, analysed for intracellular cytokine staining by FACS (top right) and transferred into irradiated recipients. The graph (bottom right) shows clinical scores for five different mice per group (mean values±s.d.). (c) Naive CD4+CD45.1+cells were stimulated with plate-bound anti-CD3/anti CD28 antibodies for the initial 72 h in Th17 differentiation conditions, in the presence or absence of WT or Jarid2 KO CD45.2+iNKTs or iNKTs + anti-IL-4, as indicated. Cells were restimulated with PMA/ionomycin and cytokine production was measured by intracellular staining. Histogram (right) represents flow cytometry analysis of the CD45.1+subset. Figure 6: Even a small contamination with Jarid2-deficient iNKT cells compromises Th17 differentiation. ( a ) Jmj fl/fl or Jmj fl/fl CD4Cre mice were immunized on day 0 with MOG(35–55) peptide in complete Freund’s adjuvant (CFA) and pertussis toxin (PTX) was administered intraperitoneally on days 0 and 1. Mice were monitored for neurological signs of EAE. Disease incidence in two combined independent experiments (middle panel); clinical scores (mean values±s.d.) in one representative experiment with at least four mice per group (right panel) are displayed. EAE disease scores were analysed by two way analysis of variance. ** P <0.01, * P <0.05. ( b ) CD4 + CD62L hi , CD44 lo (naive) T cells were isolated from 2D2 TCR-transgenic mice specific for MOG(35–55) peptide and stimulated in Th17-biasing conditions (IL-1β, IL-6 and IL-23) for 5 days. Cells were restimulated with plate-bound anti-CD3/anti-CD28 antibodies, analysed for intracellular cytokine staining by FACS (top right) and transferred into irradiated recipients. The graph (bottom right) shows clinical scores for five different mice per group (mean values±s.d.). ( c ) Naive CD4 + CD45.1 + cells were stimulated with plate-bound anti-CD3/anti CD28 antibodies for the initial 72 h in Th17 differentiation conditions, in the presence or absence of WT or Jarid2 KO CD45.2 + iNKTs or iNKTs + anti-IL-4, as indicated. Cells were restimulated with PMA/ionomycin and cytokine production was measured by intracellular staining. Histogram (right) represents flow cytometry analysis of the CD45.1 + subset. Full size image EAE can be mediated in adoptive transfer models by myelin-specific T cells of Th1 or Th17 phenotypes [52] . To investigate the protective effect associated with Jarid2 deficiency, we crossed 2D2 TCR transgenic mice, which bear a TCR specific for a MOG peptide spanning amino acids 35–55 (MOG35–55), to Jmj fl/fl and Jmj fl/fl CD4Cre mice. We then evaluated the ability of naive CD4 + T cells to differentiate into Th17 cells in vitro , and the ability of the resulting Th17 cells to induce neuroinflammation in irradiated recipient mice ( Fig. 6b ). Highly purified Jarid2-deficient naive T cells (isolated to >99% purity by sorting for CD8 − B220 − CD4 + CD25 − CD44 lo CD62L hi cells) showed no defect in IL-17A or IFN-γ production compared with WT cells when differentiated under Th17 polarizing conditions ( Fig. 6b , top right). Similarly, on transfer into irradiated B6 recipient mice, Th17 cells derived from Jarid2-deficient Jmj fl/fl CD4Cre 2D2 and control Jmj fl/fl 2D2 mice showed no significant difference in their ability to induce EAE in the recipient mice ( Fig. 6b , bottom right). Thus the absence of Jarid2 does not compromise Th17 differentiation, in agreement with a recent report [53] . Together, these results showed that compared to control mice, mice that lack Jarid2 in T cells show decreased EAE after direct immunization, whereas mice adoptively transferred with Jarid2-deficient versus control 2D2 Th17 cells showed equivalent development of disease. One possibility was that this discrepancy reflected the presence of NKT cells in the first model. To test this hypothesis, we mixed responder B6 naive CD4 + T cells (CD45.1 + ) with purified CD1d- αGalCer tetramer + iNKT cells (see Methods) from WT or Jarid2-deficient mice (CD45.2 + ) in a 99:1 ratio, activated and cultured them under Th17 conditions in vitro , and measured IL-17A production by restimulated cells on day 5 ( Fig. 6c , left). Remarkably, the presence of this minute fraction (1%) of Jarid2-deficient iNKT cells in the cultures diminished IL-17 production substantially, whereas the presence of similar numbers of WT ( Jmj fl/fl ) cells had no effect ( Fig. 6c , middle). The suppressive effect of the iNKT cells was mediated through IL-4 production, as the addition of neutralizing antibodies to IL-4 during Th17 differentiation abrogated the suppressive effect of iNKT cells on IL-17 expression ( Fig. 6c , right). Taken together, these data indicate that IL-4 produced by Jarid2-deficient iNKT cells diminishes Th17 differentiation in vitro and autoimmune pathology in vivo . Although the protective effects of Jarid2 deficiency observed in unmanipulated mice ( Fig. 6a ) are likely to be due to the ability of the expanded iNKT cell population to compromise Th17 cell differentiation in vivo , other T-cell populations that arise from DP precursors may also play an important role. Jarid2 binds at the Zbtb16 locus and regulates H3K9me3 As most of the phenotypes we observed in the thymus and periphery of Jmj fl/fl CD4Cre mice seemed to be due to the presence of an expanded PLZF hi immature iNKT cell population, we tested the hypothesis that Jarid2 is a negative regulator of PLZF (Zbtb16) in T cells. Jarid2 is a component of PRC2, which generates H3K27me3; it also interacts with the G9a-GLP complex responsible for H3K9me1/me2 and the SETDB1 complex responsible for H3K9me2/me3 (refs 13 , 15 ). We asked whether Jarid2 occupied and regulated histone modification in the PLZF (Zbtb16) locus in DP thymocytes, the precursors of iNKT cells. Jarid2 was efficiently deleted, and levels of PLZF (Zbtb16) mRNA were substantially increased, in DP thymocytes from Jmj fl/fl CD4Cre mice ( Fig. 7a ). Egr2 can directly bind and activate the PLZF (Zbtb16) promoter [29] ; however, we did not observe significant differences in Egr2 mRNA levels in total DP thymocytes ( Fig. 7b , left) or in CD69 + DP thymocytes that had undergone positive selection ( Fig. 7b , right). Thus, Jarid2 does not suppress PLZF expression indirectly by altering the transcription of Egr2 . 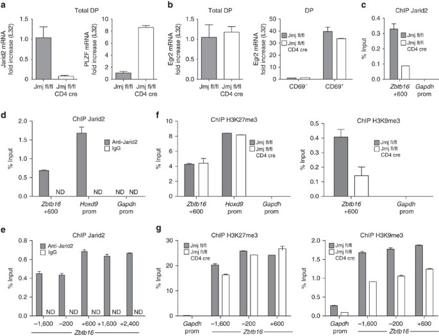Figure 7: Analyses of Jarid2 binding and histone modifications in theZbtb16promoter. Total DP (CD4+CD8+) thymocytes (a,b(left) andc–g) or DP CD69−(pre-positive selection) and CD69+(post-positive selection) (b(right)) were obtained by FACS sorting fromJmj fl/florJmj fl/fl CD4Cremice. Real-time qRT–PCR was performed for PLZF, Egr2 and Jarid2, as indicated. (c) ChIP was performed using anti-Jarid2 antibody and primers specific for the indicated positions of thePLZF (Zbtb16)locus and theGAPDHpromoter. (d) ChIP analysis was performed using anti-Jarid2 antibody or nonspecific control IgG and primers specific for the indicated positions of thePLZF (Zbtb16)locus and theGAPDH or HoxD9promoters. (e) An independent ChIP experiment using anti-Jarid2 antibody or IgG and primers specific for indicated positions atZbtb16locus. (f) ChIP analysis was performed using anti-H3K27me3 or anti-H3K9me3 antibodies, and primers specific for the indicated positions of thePLZF (Zbtb16)locus and theGAPDH or HoxD9promoters. (g) An independent ChIP experiment using anti- H3K27me3 or anti-H3K9me3 antibodies, and primers specific for the indicated positions of thePLZF (Zbtb16)locus. All experiments were repeated at least twice. Error bars show mean of PCR triplicates and s.e.m. Figure 7: Analyses of Jarid2 binding and histone modifications in the Zbtb16 promoter. Total DP (CD4 + CD8 + ) thymocytes ( a , b (left) and c – g ) or DP CD69 − (pre-positive selection) and CD69 + (post-positive selection) ( b (right)) were obtained by FACS sorting from Jmj fl/fl or Jmj fl/fl CD4Cre mice. Real-time qRT–PCR was performed for PLZF, Egr2 and Jarid2, as indicated. ( c ) ChIP was performed using anti-Jarid2 antibody and primers specific for the indicated positions of the PLZF (Zbtb16) locus and the GAPDH promoter. ( d ) ChIP analysis was performed using anti-Jarid2 antibody or nonspecific control IgG and primers specific for the indicated positions of the PLZF (Zbtb16) locus and the GAPDH or HoxD9 promoters. ( e ) An independent ChIP experiment using anti-Jarid2 antibody or IgG and primers specific for indicated positions at Zbtb16 locus. ( f ) ChIP analysis was performed using anti-H3K27me3 or anti-H3K9me3 antibodies, and primers specific for the indicated positions of the PLZF (Zbtb16) locus and the GAPDH or HoxD9 promoters. ( g ) An independent ChIP experiment using anti- H3K27me3 or anti-H3K9me3 antibodies, and primers specific for the indicated positions of the PLZF (Zbtb16) locus. All experiments were repeated at least twice. Error bars show mean of PCR triplicates and s.e.m. Full size image ChIP assays showed that Jarid2 bound the region around position +600 in the PLZF (Zbtb16) locus in DP cells ( Fig. 7c,d ), consistent with previous studies showing the presence of H3K27me3 in this region in DP thymocytes [19] , [54] . There was essentially no recovery of DNA when the chromatin was immunoprecipitated using nonspecific IgG as control ( Fig. 7d ). As a positive control, we confirmed Jarid2 occupancy of the Hoxd9 promoter ( Fig. 7d ), a well-established target of the polycomb complex [55] . Further analyses showed that Jarid2 binds a very broad region of the Zbtb16 locus, being present in all the analysed positions from −1,600 to +2,400 ( Fig. 7e ), and that H3K27me3 levels did not change between Jmj fl/fl and Jmj fl/fl CD4Cre mice at the Zbtb16 locus compared with the control ( Fig. 7f,g , left panels). In contrast, H3K9me3 levels were markedly reduced in Jarid2-deficient compared with control cells (reduction of around 37% at position +600; 47% at −200 and 50% at −1,600) ( Fig. 7f,g , right panels). Taken together, these data suggest that Jarid2 binds to the Zbtb16 locus and negatively regulates PLZF expression through controlling the deposition of H3K9me3. We show here that Jarid2, a component of both the PRC2 H3K27 methyltransferase and two different H3K9 methyltransferase (GLP-G9a and SETDB1) complexes [13] , [15] , [56] , is critical for the proper development of iNKT cells. On conditional deletion of Jarid2 in T cells ( Jmj fl/fl CD4Cre mice), iNKT cells display either a developmental arrest or skewed differentiation as discussed below. We show that these altered iNKT cell characteristics influence the development and function of other T-cell subsets in the thymus and periphery. Specifically, we document an increase of innate CD8 + T cells in the thymus of Jmj fl/fl CD4Cre mice, and also show that the presence of a very small fraction of iNKT cells impairs the ability of naive CD4 + T cells from Jmj fl/fl CD4Cre mice to differentiate into Th17 effector subsets in vitro and presumably to induce autoimmune disease in an EAE mouse model in vivo. If we use the maturation model, iNKT cells in Jarid2 -deficient mice remain at stages 1 and 2 of iNKT development and do not fully mature to stage 3 either in the thymus or in peripheral organs, as judged by low expression of CD44, negligible expression of NK1.1, CD4 expression by a high proportion of cells, high PLZF expression and increased ability to produce IL-4. According to this model, the expansion of iNKT cells in the periphery of Jmj fl/fl CD4Cre mice would reflect the higher propensity of stage 1 and 2 iNKT cells to proliferate, compared with stage 3 iNKT cells [57] . In the alternate model, the expanded iNKT cells in Jarid2-deficient mice represent NKT2-lineage cells according to a newly proposed classification of iNKT cells into NKT1 (Tbet hi ), NKT2 (GATA3 hi ) and NKT17 (RORγ hi ), respectively [45] , [48] . NKT2 cells also show high CD4 and PLZF expression and increased ability to produce IL-4 compared with NKT17 (PLZF intermediate ) and NKT1 (PLZF low ) cells [45] , [48] . Thus, depending on the model, the expanded population of iNKT cells in Jmj fl/fl CD4Cre mice could be classified as immature stage 2 iNKT cells or as NKT2 cells. iNKT cells in Jarid2-deficient mice expressed high levels of PLZF, a transcription factor that specifies both early and late stages of NKT lineage differentiation and is a key determinant of iNKT cell development and function [26] , [27] . PLZF is in turn upregulated by the transcription factor Egr2, which similar to Jarid2 is induced by TCR stimulation via the calcium/calcineurin/NFAT pathway [29] . Engagement of the homophilic SLAM family receptor Ly108 amplifies TCR signalling, increasing Egr-2 expression and consequently the expression of PLZF [58] . Notably, Egr2 mRNA levels were not altered in Jarid2-deficient relative to WT DP thymocytes, suggesting that Jarid2 represses PLZF expression by a mechanism that does not involve Egr2 . Indeed, Jarid2 directly occupies the PLZF (Zbtb16) locus in DP thymocytes and regulates H3K9me3 modification as discussed below. Nevertheless, our data suggest that Egr2 is the major positive determinant of PLZF (Zbtb16) expression, with Jarid2 having a subsidiary suppressive role. Jarid2 mRNA levels are increased after positive selection and remain high at early and late stages of iNKT maturation. Immature iNKT cells, however, express high levels of PLZF [26] , [27] as well as Egr2 (ref. 59 ), which suggests that at least at the first stages of iNKT cell maturation, Egr2 plays the predominant role in PLZF regulation. The levels of PLZF are normally downregulated in mature iNKT cells [26] , [27] ; thus, we propose that Jarid2 is a negative regulator of PLZF, and that the ability of Jarid2 to fine-tune the expression of PLZF facilitates the proper timing of iNKT cell maturation. Finally, the ability of Jarid2 to keep the PLZF (Zbtb16) locus silenced in conventional T cells may be important to restrict the number or frequency of cells that will acquire innate properties. Jarid2 associates with two distinct methyltransferase complexes that deposit ‘repressive’ histone marks, H3K27me3 deposited by Ezh2 in the PRC2 complex [8] , [9] , [10] , or H3K9me1 and me2 deposited by G9a in the G9a-GLP complex [13] . Interestingly, PRC2 and G9a/GLP physically and functionally interact to ensure epigenetic gene silencing at certain chromatin regions [60] . At a genome-wide level, Jarid2 and PRC2 bind to a largely overlapping set of target genes in mouse ESC cells, with Jarid2 seemingly required for efficient binding of PRC2 to its target loci [7] , [8] , [9] , [10] , [11] . Jarid2 contributes to mammalian PRC2 recruitment to its target genes through interaction with long non-coding RNAs [61] ; however, Jarid2-deficient ESC cells do not show genome-wide derepression of polycomb target genes, as seen in cells lacking Eed, Ezh2 and Suz12 (ref. 56 ). Moreover, in mouse ESC cells, bulk K27me3 levels are variably altered in the absence of Jarid2 (reviewed by ref. 62 ), suggesting that Jarid2 is either an optional component of PRC2, or that the functions of Jarid2 in the PRC2 complex are masked by compensatory effects, for instance from Ezh1 (ref. 63 ). In addition, Jarid2 has been reported to stimulate the H3K9 methyltransferase activity of the G9a-GLP complex in vitro [13] and also promote the recruitment of this complex to the cyclinD1 promoter in fibroblasts [13] , potentially explaining the repression of cyclinD1 by Jarid2 and the consequent effects of Jarid2 deficiency on cardiomyocyte proliferation in the heart [64] . Moreover, the failure to properly regulate Notch1 signalling was proposed to be the explanation for defects in the development of the ventricular chamber in Jarid2 mutant mice [65] . Jarid2 directly binds the SETDB1 methyltransferase and recruits it to the Notch1 locus; thus, the absence of Jarid2 results in decreased methylation of H3K9 at this locus and persistent expression of Notch1, which could explain the developmental problems in the Jarid2-deficient heart [15] . In this study, we observed that H3K9me3 levels at several regions of the Zbtb16 locus were decreased in Jarid2-deficient cells without any striking alterations in the levels of H3K27me3, supporting a preferential association of Jarid2 with H3K9 methylation in the T-cell lineage. Several strains of gene-disrupted mice show an expansion of ‘innate CD8 + T cells’ that behave similar to memory T cells as judged by their rapid production of high levels of IFN-γ in response to stimulation [66] . A common feature of these mice is the expansion of one or more subsets of PLZF + cells, which in turn drive the expansion of the innate CD8 + T cells in a cell-extrinsic manner. The mice exhibiting this phenotype can be classified into two groups: mice with impairments in T-cell signalling, such as those lacking the Tec kinases Itk or Rlk [35] , [67] , or bearing the Y145F mutation in the scaffold protein SLP-76 (ref. 38 ); and mice lacking transcriptional regulators of various kinds, including the transcription factor Klf2 (refs 39 , 40 ), the histone acetyltransferase CBP [41] , the E protein inhibitor Id3 (refs 42 , 68 ) and in this study, Jarid2. Together, the similar phenotypes of these different mouse strains define a network of diverse effector proteins involved in a pathway of TCR signalling to gene expression, which together specify increased expression of PLZF. Dissecting the role of Jarid2 in mice that exhibit enhanced development of innate CD8 + innate-like lymphocytes will be an important step in understanding the signalling events and transcriptional networks regulating the development of PLZF+ thymocytes. Mice Jmj fl/fl mice [36] , Itk−/− mice [67] , Nfat1 −/− mice [69] , Nfat2 fl/fl CD4Cre mice generated in our laboratory [70] and 2D2 transgenic mice expressing a TCR specific for the myelin oligodendrocyte (MOG35–55) peptide [71] have been described previously. For generation of mice with T cell-specific disruption of Jarid2, CD4Cre transgenic mice (Jackson) were bred with Jmj fl/fl mice and the progeny were intercrossed. 2D2 transgenic mice were also intercrossed to Jmj fl/fl CD4Cre mice. C57BL/6 (CD45.2 + ) mice, B6.SJL- PtprcaPep3bBoyJ (CD45.1 + ) and B6.PL-Thy1 a /CyJ (Thy 1.1 + ) mice were from the Jackson Laboratory. For all experiments, we used males or females of age 4 to 8 weeks old. We did not observe any phenotypic differences between males or females for the assays we performed. All breeding and experiments were reviewed and approved by the Institutional Animal Care and Use Committee of the La Jolla Institute of Allergy and Immunology. Ex vivo cell analyses by flow cytometry Cells from the thymus, spleens and lymph nodes were isolated and stained with antibodies to mouse lymphocyte surface antigens purchased from Biolegend or eBioscience, or αGalCer/CD1d tetramer (Kirin) for Vα14 i NKT cells identification. For PLZF intracellular analyses, cells were surface-stained and then stained with 2 μg ml −1 of anti-PLZF (Santa Cruz) using the Foxp3 Fixation/Permeabilization kit (eBioscience) and analysed by flow cytometry on Fortessa. Lungs and livers were collected from perfused mice, mononuclear cells were prepared by Percoll (GE Healthcare) gradient, stained and analysed for surface markers. For analyses of IL-4 and IFN-γ production, thymocytes were isolated and plated at 1 × 10 6 cells per ml. Cells were stimulated with 50 ng ml −1 PMA and 1.5 μM ionomycin (Sigma-Aldrich) for 5 h with Brefeldin A (10 μg ml −1 ) added for the final 3 h. Surface marker staining was performed, followed by intracellular cytokine staining. For intracellular staining, cells were washed in PBS–1% BSA, fixed with 2% paraformaldehyde in PBS for 15 min at 4 °C, washed in PBS, permeabilized in saponin buffer (PBS, 0.5% saponin (Sigma) and stained with 2 μg ml −1 anti-IL-4 or anti-IFN-γ (eBioscience). For enrichment of iNKT cells from thymocytes, CD8α + , TER-119 + and CD19 + cells were excluded using Dynabeads (Invitrogen). Depleted samples were stained using αGalCer/CD1d tetramer, TCRβ, CD44 and NK1.1 (gating strategy in Fig. 3h , top), and sorted on FACSAria II. iNKT cell culture and activation iNKTs, purified as described above, were cultured in the presence of bone marrow-derived dendritic cells (DCs) pulsed with αGalCer (and irradiated at 500 rads) for 3 days. Activated iNKTs were expanded for 14 days in the presence of mIL-7 (10 ng ml −1 ). ‘Rested’ iNKTs were TCR activated by plate bound anti-CD3 (3 μg ml −1 ) and anti-CD28 (1 μg ml −1 ) for indicated times and gene expression was analysed by qPCR. CD4 + T cell differentiation and stimulation CD4 + BB20 − CD8 − CD25 − CD62L hi CD44 lo T cells were FACS sorted from lymph nodes and spleens of 5- to 8-week-old mice and activated with plate bound anti-CD3 and anti-CD28 antibodies at 1 μg ml −1 in the presence of 10 μg ml −1 of anti-IL4, 20 ng ml −1 of IL-1β, 20 ng ml −1 of IL-6 and 50 ng ml −1 of IL-23 (Th17 conditions). Cells were counted and replated at 0.5 × 10 6 cells per ml on days 3 and 4 after initial stimulation. Cyclosporin A (Calbiochem 239835) was added to a final concentration of 2 μM. On day 5, differentiated cells were restimulated with PMA (10 nM) and ionomycin (1 μM) for 5 h. Brefeldin A (10 μg ml −1 ) was added during the last 2 h of stimulation. Intracellular staining was performed as described in ‘ Ex vivo cell analyses by flow cytometry’ and the anti-IL-17A antibody (eBioscience) was used at 2 μg ml −1 . For the experiment with ‘modifiers’ iNKT, 99% of CD4 + BB20 − CD8 − CD25 − CD62L hi CD44 lo T cells FACS sorted from lymph nodes and spleens of B6.SJL-PtprcaPep3bBoyJ (CD45.1+) mice were mixed with 1% of BB20 − CD8 − CD25 − CD62L lo CD44 hi TCRβ + αGal-Cer tetramer + FACS sorted from lymph nodes and spleens of Jmj fl/fl or Jmj’fl/fl CD4Cre mice. The mixed populations were stimulated under Th17 polarizing conditions in the presence or absence of 1 μg ml −1 of anti-IL-4 (from NCI). Mixed bone marrow chimeras T cell-depleted precursors cells were obtained by excluding CD3ε + cells (using MACS Anti-Biotion Microbeads (Miltenyi Biotec)) from bone marrow derived from CD45.2 + ( Jmj fl/fl or Jmj fl/fl CD4cre mice) or CD45.1 + (B6.SJL) mice. CD45.2 + and CD45.1 + cells were mixed in equal ratios (1:1) and cells were transferred to lethally irradiated (1,000 rads) Thy1.1 + host animals. Chimeras were analysed 9 weeks after the transplant. Single-cell suspensions of thymus were analysed by flow cytometry. EAE induction For the induction of EAE, Jmj fl/fl or Jmj fl/fl CD4Cre mice were immunized with MOG peptide emulsified in complete Freund’s adjuvant. Mice were immunized subcutaneously at the dorsal flanks with 150 μg of MOG peptide in complete Freund’s adjuvant at day 0. Pertussis toxin was given intraperitoneally at day 1 and day 2 with the dosage of 200 ng per mouse. Naive CD4 + T cells isolated from 2D2 TCR-transgenic mice were skewed under Th17 conditions. On day 5 after initial activation, cells were harvested and restimulated with plate-bound anti-CD3 and anti-CD28 at 1 μg ml −1 in the presence of IL-2 (20 units per ml) and IL-18 (25 ng ml −1 ) for 16–18 h. Subsequently, the cells were harvested, washed with PBS and one- to two million cells were transferred intraperitoneally into lightly irradiated (400 rads) 6- to 8-week-old recipient B6 mice [52] . Animals were monitored daily for development of EAE according to the following criteria: 0, no disease; 1, decreased tail tone; 2, hind limb weakness or partial paralysis; 3, complete hindlimb paralysis; 4, front and hind limb paralysis; 5, moribund state. In addition, the body weight of the mice was measured during each clinical assessment. Chromatin immunoprecipitation FACS-sorted DP cells were fixed for 10 min with 1% formaldehyde at room temperature at 1 × 10 7 cells per ml. Fixation was stopped with 120 mM glycine for 5 min. Fixed cells were washed 2 × with cold PBS. After washes, nuclei were obtained and chromatin (40 × 10 6 cell equivalents) was sheared with Covaris to yield 200–500 bp DNA fragments. Sheared chromatin were immunoprecipitated overnight at 4 °C using protein G Dynabeads coated with anti-Jarid2 Catalog# NB100-2214 (Novus Biologicals, Littleton, CO), anti-H3K27me3 or H3K9me3 (Abcam). A total of 20–40 × 10 6 cells were used for each Jarid2 ChIP and 2–5 × 10 6 for histone modification ChIP analyses. Both input and ChIP DNA were then treated with RNase A (5 μg total) for 1 h at 37 °C, followed by addition of Proteinase K (5 μg total) and overnight incubation at 65 °C to reverse cross-linking. DNA was then purified with QIAquick columns (QIAGEN Gel Extraction Kit) as per the manufacturer’s instructions and resuspended in a 50-μl volume. For real-time PCR detection of immunoprecipitated targets using the Roche SYBR green real-time master mix, a standard curve was obtained with serial dilutions of input DNA for each sample and 2 μl ChIP DNA was used per PCR reaction. Sequences of primers used for the qPCR showed in Supplementary Table 1 . Quantitative real-time reverse transcription PCR Total RNA from CD4 + T cells, total DPs, CD69 − or CD69 + DPs was prepared using RNeasy PLUS kit (Qiagen). Complementary DNA was synthesized using Superscript reverse transcriptase and oligo(dT) primers (Invitrogen), and gene expression was examined with Step One Plus (Applied Biosystems) using Roche SYBR green real-time master mix. Sequences of primers used for the qPCR showed in Supplementary Table 1 . Statistical analysis Statistical analysis, unpaired t -tests or two-way analysis of variance were performed with Prism (Graphpad Software), and the P -values are indicated for each figure. P -values <0.05 were considered nonsignificant. How to cite this article: Pereira, R. M. et al . Jarid2 is induced by TCR signalling and controls iNKT cell maturation. Nat. Commun. 5:4540 doi: 10.1038/ncomms5540 (2014).